Continuous electroproduction of formate via CO2reduction on local symmetry-broken single-atom catalysts Atomic-level coordination engineering is an efficient strategy for tuning the catalytic performance of single-atom catalysts (SACs). However, their rational design has so far been plagued by the lack of a universal correlation between the coordination symmetry and catalytic properties. Herein, we synthesised planar-symmetry-broken CuN 3 (PSB-CuN 3 ) SACs through microwave heating for electrocatalytic CO 2 reduction. Remarkably, the as-prepared catalysts exhibited a selectivity of 94.3% towards formate at −0.73 V vs. RHE, surpassing the symmetrical CuN 4 catalyst (72.4% at −0.93 V vs. RHE). In a flow cell equipped with a PSB-CuN 3 electrode, over 90% formate selectivity was maintained at an average current density of 94.4 mA cm −2 during 100 h operation. By combining definitive structural identification with operando X-ray spectroscopy and theoretical calculations, we revealed that the intrinsic local symmetry breaking from planar D 4 h configuration induces an unconventional dsp hybridisation, and thus a strong correlation between the catalytic activity and microenvironment of metal centre (i.e., coordination number and distortion), with high preference for formate production in CuN 3 moiety. The finding opens an avenue for designing efficient SACs with specific local symmetries for selective electrocatalysis. Formic acid has long been regarded as an important liquid feedstock for valuable chemicals synthesis and ideal hydrogen carrier material owing to its high volumetric (53.4 g L −1 ) and moderate gravimetric (4.4 wt%) hydrogen storage capacity in ambient conditions [1] , [2] . Producing formic acid via the electrochemical reduction of carbon dioxide (CO 2 ) is therefore attracting widespread attention [3] , [4] , [5] . Considering both the thermodynamical and kinetic energy barriers, the energy consumption for electroreduction of CO 2 to formic acid ( \({{{{{\rm{C}}}}}}{{{{{{\rm{O}}}}}}}_{2}+2{{{{{{\rm{H}}}}}}}^{+}+2{{{{{{\rm{e}}}}}}}^{-}\to {{{{{\rm{HCOOH}}}}}}\) , −0.19 V vs. RHE) is relatively less compared with other products like CH 3 OH and CH 4 . In the past years, various metals (e.g., Cu, Sn, Bi) and their alloys have been prepared as electrocatalysts for electrocatalytic CO 2 to formic acid [6] , [7] , [8] , [9] , [10] . Although significant progress has been made in reducing the overpotential for CO 2 electroreduction to formic acid [11] , [12] , [13] , [14] , achieving the necessary faradaic efficiency (FE) and current density for practical applications remains a challenge [15] , [16] , [17] . Hence, there is a pressing demand to develop highly selective and energy-efficient catalysts for the electroreduction of CO 2 to formic acid. Carbon-supported single-atom catalysts (SACs), most of which usually adopt a prototypical MN 4 moiety with local planar-like D 4 h symmetry, show great promise for accelerating the kinetics of heterogeneous catalysis owing to their unique physicochemical properties [18] , [19] , [20] . Though substantial progress has been made in activity improvement, recent studies reveal that the highly symmetrical MN 4 architecture actually imposes serious limitations on the electronic configuration regulation of the active metal site [21] , [22] , [23] . To lift the confinement and better tune the electronic structures of the active sites, various coordination engineering strategies such as tuning the coordination species and the coordination number of the active centres, heteroatom substitution, neighbouring metal interactions are developed [24] , [25] , [26] , [27] . For example, the coordination-engineered M-N x /N x L y (L=C, O, P, S) exhibits excellent performance in oxygen-involved electrocatalysis with a medium bond strength (494 kJ mol −1 for O=O bond) [23] , [28] , [29] , [30] , [31] , [32] , [33] , and great potentials for activating the molecules with high bond energy such as C=O in CO 2 (750 kJ mol −1 ) [34] , [35] , [36] , [37] , [38] , [39] . Essentially, local symmetry breaking from the planar-like D 4 h via coordination engineering can redistribute the electronic (anti-)bonding states on specific d / s / p orbitals of the metal sites along with the energy scale and thereby maximumly regulate their hybridisation interaction in a rationally pre-selected local symmetry. This local symmetry manipulation could thus facilitate the adsorption and activation of CO 2 molecular as well as reactive intermediates and optimise the reaction pathways for CO 2 reduction reaction (CO 2 RR) with high activity and selectivity [40] . Unfortunately, except for the extrinsic addition of various axial ligands, there is no report about the intrinsic local symmetry breaking in M-N x SACs for electrocatalytic CO 2 reduction to date. Moreover, despite the extensive endeavours, the underlying mechanism that governs the structure−functionality relationship and the universal design principle to manipulate the local coordination symmetry remains unclear. Herein, the local planar-symmetry-broken CuN 3 (PSB-CuN 3 ) SACs were synthesised by a facile and simple microwave process for electroreduction of CO 2 . The as-prepared PSB-CuN 3 delivers a selectivity of 94.3% for electroreduction of CO 2 into formate at a potential of −0.73 V vs. RHE, which outperforms the CuN 4 SACs with local planar D 4 h symmetry (PS-CuN 4 ) with a maximum selectivity of 72.4% at a given potential of −0.93 V vs. RHE. Impressively, the flow cell equipped with the PSB-CuN 3 electrode exhibits over 90% formate selectivity at an average reduction current density of 94.4 mA cm −2 during 100 h continuous operation at an applied potential of −0.95 V vs. RHE. By combining definitive structural identification with ex-situ/operando X-ray spectroscopy characterisations and systematic theoretical calculations, we reveal that the intrinsic local symmetry breaking from the planar-like D 4 h to C 2 v configuration induces an unconventional dsp hybridisation. It causes the catalytic activity unconformable to the widely used d -band centre theory, but strongly correlated with the local environment of the metal centre (i.e., coordination number and geometric distortion), which can serve as a universal descriptor to predict the activities of H 2 /CO/HCOOH productions for graphene-based SACs, with a high preference for formate production in CuN 3 moiety. Synthesis and structural characterisation of PSB-CuN 3 catalyst PSB-CuN 3 is synthesised via a microwave heating strategy, as schematically illustrated in Fig. 1a . Amine-functionalised graphene nanosheets (AGNs) are used to immobilise the Cu 2+ ions through an electrostatic interaction. Then, PSB - CuN 3 is obtained through a rapid microwave heating process within five seconds. In comparison to conventional thermal annealing, microwave-induced instant heating leads the local environment in the material to change dramatically, facilitating the formation of a local symmetry-breaking architecture. The ultrathin morphology of as-synthesised PSB-CuN 3 can be discerned well by transmission electron microscopy (TEM) and high-angle annular dark-field scanning TEM (HAADF-STEM) images, in which the edges of the two dimentional (2D) nanosheets spontaneously curl upon microwave heating (Fig. 1b, c , Supplementary Fig. 1a ). The aberration-corrected HAADF-STEM (AC-HAADF-STEM) image (Supplementary Fig. 1b ) shows that no Cu-derived nanoparticles can be observed, which agrees with the X-ray diffraction (XRD) result (Supplementary Fig. 2 ). Meanwhile, the atomic dispersion of single Cu atoms can be directly identified as the obvious individual bright dots in the high-magnification AC-HAADF-STEM images (Fig. 1d, e ). Energy-dispersive X-ray spectroscopy (EDS) mappings analysis shows C, N and Cu elements are homogeneously dispersed on the entire architecture of PSB-CuN 3 (Fig. 1f ) with a content of 96.7 at %, 2.82 at % and 0.48 at %, respectively (Supplementary Fig. 3 ). And, the atomic force microscopy (AFM) measurement (Fig. 1g ) is performed to present the average thickness of the PSB-CuN 3 (~1.61 nm). The N 2 adsorption-desorption isotherms shows a high specific surface area of ~510 m 2 g −1 with dominant pore sizes of ~4 nm (Supplementary Fig. 4 ). The PS-CuN 4 catalyst prepared by conventional thermal annealing shows similar physiochemical information (Supplementary Figs. 2 – 6 ), demonstrating the high controllability for materials synthesis. Subsequently, chemical states of the elements in PSB-CuN 3 and PS-CuN 4 are investigated by X-ray photoelectron spectroscopy (XPS) analysis (Supplementary Figs. 7 – 9 ). While three types of graphitic (401.2 eV), pyrrolic (399.4 eV) and pyridinic (398.6 eV) N species for stabilising the Cu atoms exhibit no obvious difference, the Cu 2 p spectrum of PSB - CuN 3 possesses two dominant peaks at binding energies of 932.0 eV (2 p 3/2 ) and 951.8 eV (2 p 1/2 ) that are obviously lower than the characteristic binding energies of 934.3 and 954.1 eV for the Cu 2+ in PS-CuN 4 , implying a lower valence state of Cu 1+ in PSB - CuN 3 . Cu LMM spectra are obtained to further demonstrate the chemical valence of the two samples (Supplementary Fig. 10 ). While PSB-CuN 3 is dominated by Cu 1+ species located at 571.1 eV, PS-CuN 4 is dominated by Cu 2+ species located at 572.0 eV [41] . In addition to the chemical states, Raman spectra show there are a larger number of structural defects in PSB-CuN 3 compared with PS-CuN 4 (Supplementary Fig. 11 ). Thus, the above results suggest that the Cu species in PSB - CuN 3 catalyst are likely to be dispersed as unusual low-valent mononuclear centres on largely defective graphene nanosheets. Fig. 1: Synthesis and structural characterisations of PSB-CuN 3 catalyst. a Schematic illustration of the preparation strategy for PSB-CuN 3 and PS-CuN 4 . b – e TEM image ( b ; scale bar, 200 nm), HAADF-STEM image ( c scale bar, 200 nm), AC-HAADF-STEM image ( d scale bar, 1 nm) and corresponding intensity maps ( e ) of PSB-CuN 3 . f EDS mapping images of PSB-CuN 3 (C, red; N, orange; Cu, blue; scale bar, 10 nm). Note that the molybdenum grid was used for all STEM measurements. g AFM image of as-prepared PSB-CuN 3 (scale bar, 2 μm), showing measured dimensions of individual nanosheets. Full size image Atomic and electronic structure analysis of PSB-CuN 3 catalyst by X-ray absorption fine structure spectroscopy The coordination environment and chemical state of PSB-CuN 3 are further explored by element-selective X-ray absorption fine structure (XAFS) spectroscopy analysis including extended-XAFS (EXAFS) and X-ray absorption near-edge structure (XANES). Figure 2a shows the Cu K -edge EXAFS Fourier-transformed (FT) magnitudes. 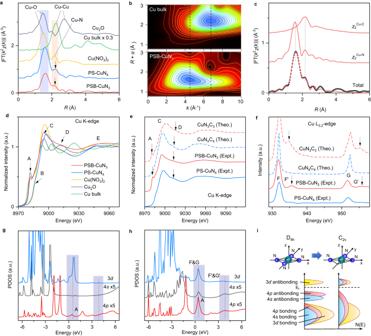Fig. 2: Atomic and electronic structure characterisation by XAFS spectroscopy. aFourier-transformed magnitudes of the experimental CuK-edge EXAFS signals of PSB-CuN3and PS-CuN4along with reference samples. The Fourier transforms are not corrected for phase shifts.bEXAFS wavelet transforms for the PSB-CuN3and reference samples. The contour maxima at ~4.2 and 7.0 Å−1(dashed lines) are associated with the Cu–N/C and Cu–Cu contributions, respectively.cCuK-edge EXAFS analysis of PSB-CuN3with the Cu–N and Cu–C two-body backscattering signalsχ2included in the fit. The calculated (red line) and measured (black dots) spectra show excellent agreement (Supplementary Table1).dExperimental CuK-edge XANES spectra of PSB-CuN3, PS-CuN4and reference samples.e,fComparison between the experimental CuK-edge (e) andL3,2-edge (f) XANES spectra of PS-CuN4and PSB-CuN3and the theoretical spectra calculated for the depicted CuN4C4and CuN3C3structures (Supplementary Fig.21).g,hThe calculated 3d, 4sand 4pprojected densities of states on the Cu sites in CuN4C4(g) and CuN3C3(h) structures.iSchematic diagrams of band shifts and hybridisation for the planar CuN4moiety with localD4hsymmetry and the defective CuN3moiety with lower local C2vsymmetry. a.u. arbitrary units. Both PSB-CuN 3 and PS-CuN 4 exhibit a major peak at ~1.60 Å and a minor satellite peak at ~2.20 Å, which is similar to the archetypical profile of pyridinic-N-based MN 4 C 4 motifs [21] . Concurrently, the EXAFS wavelet-transform analysis is performed to more clearly discriminate the coordination atoms [42] . Only one intensity maximum at ~4.2 Å –1 is detected in the two catalysts (Fig. 2b ), which confirms the assignment of the major and minor peaks to the Cu–N/C bonding (Supplementary Fig. 12a ). However, the two peaks intensities in PSB-CuN 3 are obviously weaker than that in PS-CuN 4 (Supplementary Fig. 12b ), which implies a lower coordination configuration for Cu atoms in PSB-CuN 3 . Subsequently, quantitative EXAFS curve-fitting analysis is carried out to investigate the coordination configuration (Fig. 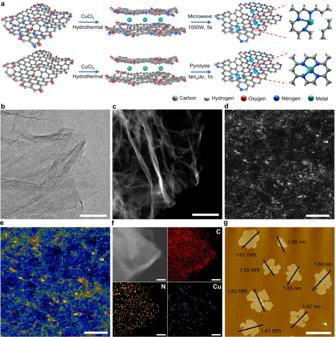2c , Supplementary Figs. Fig. 1: Synthesis and structural characterisations of PSB-CuN3catalyst. aSchematic illustration of the preparation strategy for PSB-CuN3and PS-CuN4.b–eTEM image (b; scale bar, 200 nm), HAADF-STEM image (cscale bar, 200 nm), AC-HAADF-STEM image (dscale bar, 1 nm) and corresponding intensity maps (e) of PSB-CuN3.fEDS mapping images of PSB-CuN3(C, red; N, orange; Cu, blue; scale bar, 10 nm). Note that the molybdenum grid was used for all STEM measurements.gAFM image of as-prepared PSB-CuN3(scale bar, 2 μm), showing measured dimensions of individual nanosheets. 13 – 17 ; Supplementary Table 1 ). Coordination numbers of the first N and second C coordination spheres in PS-CuN 4 are estimated to be 4.0 and 4.1 at distances of 2.00 and 2.67 Å, respectively, supporting the adoption of a pyridinic-N-based CuN 4 C 4 configuration (Supplementary Fig. 17c ). By contrast, the best-fit for PSB-CuN 3 demonstrates reduced coordination numbers (2.8 for Cu–N and 2.9 for Cu–C) with contracted interatomic distances (1.98 Å for the first Cu–N and 2.65 Å for Cu–C) for the first and second coordination spheres, suggesting a defective pyridinic-N-based CuN 3 C 3 configuration (Fig. 2c ). Fig. 2: Atomic and electronic structure characterisation by XAFS spectroscopy. a Fourier-transformed magnitudes of the experimental Cu K -edge EXAFS signals of PSB-CuN 3 and PS-CuN 4 along with reference samples. The Fourier transforms are not corrected for phase shifts. b EXAFS wavelet transforms for the PSB-CuN 3 and reference samples. The contour maxima at ~4.2 and 7.0 Å −1 (dashed lines) are associated with the Cu–N/C and Cu–Cu contributions, respectively. c Cu K -edge EXAFS analysis of PSB-CuN 3 with the Cu–N and Cu–C two-body backscattering signals χ 2 included in the fit. The calculated (red line) and measured (black dots) spectra show excellent agreement (Supplementary Table 1 ). d Experimental Cu K -edge XANES spectra of PSB-CuN 3 , PS-CuN 4 and reference samples. e , f Comparison between the experimental Cu K -edge ( e ) and L 3,2 -edge ( f ) XANES spectra of PS-CuN 4 and PSB-CuN 3 and the theoretical spectra calculated for the depicted CuN 4 C 4 and CuN 3 C 3 structures (Supplementary Fig. 21 ). g , h The calculated 3 d , 4 s and 4 p projected densities of states on the Cu sites in CuN 4 C 4 ( g ) and CuN 3 C 3 ( h ) structures. i Schematic diagrams of band shifts and hybridisation for the planar CuN 4 moiety with local D 4 h symmetry and the defective CuN 3 moiety with lower local C 2 v symmetry. a.u. arbitrary units. Full size image Due to the higher sensitivity to the 3D arrangement of atoms around the photo-absorber, XANES spectroscopy is applied to better identify the atomic-site structures [43] , [44] . Figure 2d shows the hard Cu K -edge XANES spectra for the samples along with references. The PS-CuN 4 exhibits a shoulder feature B at ~8987 eV, which is close to that of Cu(NO 3 ) 2 . It arises from the 1 s →4 p z transition of a planar-like Cu 2+ configuration [45] , [46] . However, in the spectrum of PSB-CuN 3 , a pronounced peak A is observed at a much lower energy of ~8982 eV as in Cu 2 O, signifying an unusual Cu 1+ configuration. Moreover, PSB-CuN 3 shows a more flattened profile for the post-edge features C, D and E compared with PS-CuN 4 . This tendency is also corroborated by the soft XANES results (Supplementary Figs. 18 – 20 ). And, the Cu L 3,2 -edge spectra reveal an emergence of two extra post-edge resonant peaks from PS-CuN 4 to PSB-CuN 3 that coincides with the positions of Cu 2 O (Supplementary Fig. 20 ). Those hard and soft XANES differences indicate a peculiar Cu 1+ species in PSB-CuN 3 and a planar-like Cu 2+ species in PS-CuN 4 , consistent with the XPS results (Supplementary Figs. 9 and 10 ). Then, as guided by the EXAFS results, we constructed various CuN x C y structural models with different local symmetry (Supplementary Figs. 21 and 22 ) and resorted to XANES simulation to identify the specific configuration. Figure 2 e, f shows that the CuN 4 C 4 moiety with local D 4 h symmetry (Note: The C 4 symmetry axis is perpendicular to the plane) reproduces properly the experimental K - and L 3,2 -edge XANES profiles of PS-CuN 4 . In addition, when a N defect is introduced, the obtained CuN 3 C 3 moiety shows a local symmetry breaking from D 4 h to C 2 v (Note: The remaining C 2 symmetry axis is in the plane) and it produces an excellent agreement to the experimental profiles of PSB-CuN 3 , particularly for the characteristic peaks A and D at K -edge (Fig. 2e ) and for the peaks F’ and G’ at L 3,2 -edge (Fig. 2f ). By contrast, more N defects in CuN 2 C 2 moiety lead to a dramatic discrepancy in the profiles (see Supplementary Fig. 23 ). The probability for the substitution of the N atoms in the first coordination sphere by C atoms can also be excluded (Supplementary Figs. 24 and 25 , Supplementary Table 2 and Supplementary Note 1 ). Therefore, the combination of EXAFS and XANES analyses has unambiguously revealed a dominance of defective CuN 3 C 3 moiety with lower local C 2 v symmetry and mono-valence implanted in a graphene sheet for PSB-CuN 3 catalyst. Because the K -edge (1s→4 p transition) and L 3,2 -edge (2 p →3 d transition) XANES can probe the unoccupied density of states on the 4 p and 3 d orbitals of the Cu sites, the emergent resonant features (A, F’ and G’) in PSB-CuN 3 catalyst indicate a unique p and d electronic distribution that can be regulated by the local coordination symmetry. Detailed analysis on the density of states (Fig. 2g–i , Supplementary Figs. 26 and 27 and Supplementary Note 2 ) unveils that the local symmetry lowering from D 4 h in CuN 4 C 4 to C 2 v in CuN 3 C 3 can drive an obvious upshift of the anti-bonding 4 s and 4 p state to above the Fermi energy and finally trigger a dramatic dsp hybridisation at the energy positions of peaks A/F/G and F’/G’, where the p orbital is dominated by the in-plane p x / p y orbital. The local symmetry lowering to C 2 v in CuN 2 C 2 promotes a dsp [2] hybridisation with the p orbital arising mainly from the in-plane p x and p y orbitals (Supplementary Fig. 28 and Supplementary Note 2 ). Accordingly, those anti-bonding state upshifts induced by local symmetry breaking in defective CuN x C y moieties can be pivotal to modifying the adsorption strength of the reactive intermediates and thus optimise the reaction pathways for CO 2 RR with high activity and selectivity. Evaluation of CO 2 RR performance The intrinsic CO 2 RR activity of the as-prepared samples was performed in a gas-tight H-type cell by coating a thin electrocatalyst layer on the carbon fibre paper with a catalyst loading of 0.5 mg cm −2 . The electrolytes pH (pH = 7.3 for CO 2 saturated 0.5 M KHCO 3 ) and the potential of the reference electrode were checked before the test to ensure the reliability of the as-obtained electrochemical results (Supplementary Figs. 29 and 30 ). Linear sweep voltammetry (LSV) is employed to obtain polarisation curves of PSB-CuN 3 , PS-CuN 4 and AGNs electrodes in the Ar and CO 2 saturated 0.5 M KHCO 3 aqueous solution. As shown in Supplementary Fig. 31 , the reduction current increases greatly when the electrolyte solution is saturated with CO 2 . Supplementary Fig. 32 shows a sharp increased cathode current response started at an onset potential of −0.41 V vs. RHE observed from the PSB-CuN 3 electrode. By contrast, PS-CuN 4 exhibits an onset potential (−0.72 V vs. RHE) under identical conditions. Further, chronoamperometric measurements were carried out at different potentials to quantitively identify product distributions using online gas chromatography and nuclear magnetic resonance (NMR) spectroscopy (Supplementary Figs. 33 and 34 ). As shown in Supplementary Fig. 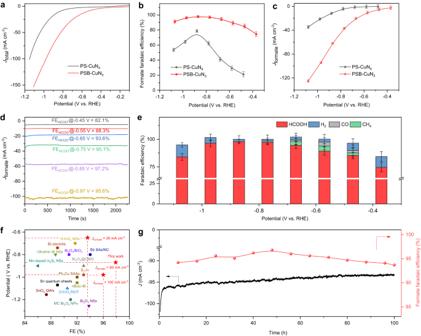Fig. 3: Evaluation of CO2RR catalytic activity by electrochemical measurements. aLinear sweep voltammetry curves of PSB-CuN3and PS-CuN4in a flow-cell setup using 0.5 M KHCO3electrolyte at 25 °C.bThe corresponding formate FEs under different potentials. The maximal formate FE of PSB-CuN3is 97.9% at −0.87 V vs. RHE.cComparison of partial current density for CO2-to-formate conversion between PSB-CuN3and PS-CuN4. The maximal formate partial current on PSB-CuN3reached 125 mA cm−2at −1.1 V vs. RHE, which represents 3.6 folds higher than that of PS-CuN4.dChronoamperometric responses of PSB-CuN3in CO2-saturated electrolyte at different potentials. The potential was corrected with 100%iRcompensation.eThe corresponding FEs of different products under different potentials on PSB-CuN3. Note that the total FEs are not complete 100% due to systems errors and double layer current of catalysts. The presented values represent the mean, while the error bars indicate the standard deviation, based on three independent measurements.fComparison of formate FEs and overpotentials for PSB-CuN3and various catalysts reported at similar conditions (See the details in Supplementary Table5).gLong-term stability test of PSB-CuN3at a potential of −0.95 V vs. RHE. 35 and Supplementary Table 3 , formate is the only liquid product from the CO 2 RR, with a certain amount of gaseous products including methane, carbon monoxide and hydrogen. No other C 1 and C 2 liquids (i.e., methanol, ethanol, n-propanol and acetone) were detected (Supplementary Fig. 34 ). Impressive FEs (HCOO − ) (>90%) were obtained with the PSB-CuN 3 throughout the potential range (−0.75 to −1.0 V vs. RHE). On the contrary, the maximal FEs of formate for PS-CuN 4 and AGNs electrodes are 72.4% and 9.5% under identical testing conditions. This suggests the PSB-CuN 3 moiety should be responsible for the high selectivity for formate. Besides, chronoamperometric measurement was carried out to investigate the stability of the as-prepared PSB-CuN 3 . As shown in Supplementary Fig. 36 , the FE of the PSB-CuN 3 electrode is ~92% after 16 h electrocatalysis compared with PS-CuN 4 (~27%). To investigate CO 2 reduction performance under industrial level current of PSB-CuN 3 , a flow cell equipped with gas diffusion electrodes (GDEs) was fabricated (Supplementary Fig. 37 ). Figure 3a shows that the GDE with PSB-CuN 3 could be operated at a current density of 150 mA cm −2 , with modest overpotentials in 0.5 M KHCO 3 solution, which is much higher than the PS-CuN 4 under the same applied potential. The optimal FEs of PSB-CuN 3 electrode is 97.9%, which is higher than the PS-CuN 4 (78.8%) (Fig. 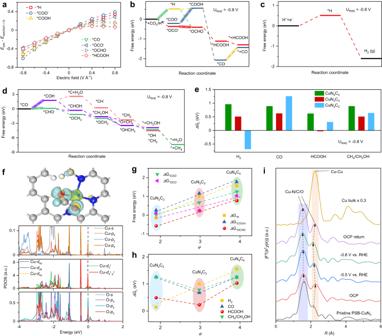Fig. 4: First-principles calculations and operando XAFS characterisation on PSB-CuN3catalysing CO2RR. aElectric field effects on the adsorbate bindings on the CuN3C3structure.b–dGibbs free-energy diagrams for CO2electroreduction to CO, HCOOH, H2, CH4and CH3OH on CuN3C3structure. The highlights indicate the potential limiting steps.eMagnitudes of the theoretical limiting free-energy differences (ΔGL) for CO, HCOOH, H2and CH4/CH3OH productions.fDifferential charge density and projected density of states for the Cu centre and the bound O atom in the adsorbed *OCHO intermediates supported on CuN3C3structure. White, grey, blue, red and cyan balls represent H, C, N, O and Cu atoms, respectively. The black dashed line represents the Femi energy level.gAdsorption free energies of ΔG*OCO−, ΔG*COO−, ΔG*OCHO, ΔG*COOHand ΔG*Hvs. the descriptorφ.hThermodynamic relations (volcano) lines for the H2, CO and HCOOH productions as a function of the descriptorφ.iFourier-transformed magnitudes of operando CuK-edge EXAFS spectra for PSB-CuN3recorded at various applied potentials vs. RHE in 0.5 M KHCO3aqueous solution. a.u., arbitrary units. 3b and Supplementary Table 4 ). With this FE, a CO 2 RR to formate partial current density of ~62 mA cm −2 was achieved (Fig. 3c ). Moreover, the FE of PSB-CuN 3 for HCOO − can be maintained over 90% through a wide applied potential range from −0.65 to −0.97 V vs. RHE (Fig. 3d, e ), exhibiting excellent selectivity for CO 2 RR-to-formate. It should be stressed that both the selectivity and activity of the PSB-CuN 3 are comparable to the previously best-reported CO 2 RR-to-HCOO − catalysts (Fig. 3f and Supplementary Table 5 ). Turnover frequency (TOF), as a key parameter for CO 2 RR efficiency assessment, is then calculated based on the standard equation. As shown in Supplementary Fig. 38 , the maximum TOF value of PSB-CuN 3 is 30825.3 h −1 at a given potential of −1.1 V vs. RHE, considerably higher than PS-CuN 4 (8558.8 h −1 ) and is comparable to the recently best-reported CO 2 RR-to-HCOO − catalysts (Supplementary Table 5 ). To show the scalability of the as-fabricated flow cell with PSB-CuN 3 electrode, the long-term durability was tested under the large current density. As shown in Fig. 3g , the PSB-CuN 3 electrode maintains an average current density of 94.4 mA cm −2 with over 90% FE formate during 100 h testing. By contrast, the PS-CuN 4 electrode shows 58.3% of the initial reduction current of 25 mA cm −2 with an average FE of 68% (Supplementary Fig. 39 ). Further structural stability characterisation by AC-HAADF-STEM and XAFS suggest that the Cu atom and its coordinating matrix in PSB-CuN 3 are robust enough to withstand the CO 2 RR operation condition (see below detailed discussion). Thus, the PSB-CuN 3 electrode could be readily incorporated into practical CO 2 RR electrolysers because of its high activity, selectivity and durability at large current densities. Fig. 3: Evaluation of CO 2 RR catalytic activity by electrochemical measurements. a Linear sweep voltammetry curves of PSB-CuN 3 and PS-CuN 4 in a flow-cell setup using 0.5 M KHCO 3 electrolyte at 25 °C. b The corresponding formate FEs under different potentials. The maximal formate FE of PSB-CuN 3 is 97.9% at −0.87 V vs. RHE. c Comparison of partial current density for CO 2 -to-formate conversion between PSB-CuN 3 and PS-CuN 4 . The maximal formate partial current on PSB-CuN 3 reached 125 mA cm −2 at −1.1 V vs. RHE, which represents 3.6 folds higher than that of PS-CuN 4 . d Chronoamperometric responses of PSB-CuN 3 in CO 2 -saturated electrolyte at different potentials. The potential was corrected with 100% iR compensation. e The corresponding FEs of different products under different potentials on PSB-CuN 3 . Note that the total FEs are not complete 100% due to systems errors and double layer current of catalysts. The presented values represent the mean, while the error bars indicate the standard deviation, based on three independent measurements. f Comparison of formate FEs and overpotentials for PSB-CuN 3 and various catalysts reported at similar conditions (See the details in Supplementary Table 5 ). g Long-term stability test of PSB-CuN 3 at a potential of −0.95 V vs. RHE. Full size image Mechanism of CO 2 activation and reduction by first-principles calculation and operando spectroscopies To understand the origin of high efficiency toward formate generation on PSB-CuN 3 catalyst, first-principles calculations were carried out for the electroreduction process of CO 2 on various graphene-based CuN x C y structures. We considered the reaction pathways for CO, formate, methanol and methane productions as well as the competing hydrogen evolution reaction (HER). For the formation of intermediate *OCHO/*COOH, two mechanisms were considered, i.e., a reaction with *H via a CO 2 insertion reaction into the metal–hydrogen bond and a direct protonation with H + from solution [47] , [48] . The optimised structures of the intermediates and the Gibbs free-energy diagrams at zero electrode potential show remarkable response to the coordination environment (Supplementary Figs. 40 – 47 , Supplementary Tables 6 and 7 ). On the CuN 4 C 4 and CuN 3 C 3 structures, the different adsorbed states of *COO − and *OCO − for CO 2 via the first electron addition are suggested to be the potential limiting steps for CO and formate productions, respectively, and the *OCO − formation is more energetically favoured than *COO − . By contrast, on the CuN 2 C 2 structure, the potential limiting steps shift to the desorption of CO and formate. The pathways initiated by *H adsorption do not show any preference than the pathways initiated by *COO − /*OCO − adsorption. It is well documented that the reduction of CO 2 to CH 4 and CH 3 OH shares similar pathways until the formation of *CO intermediate, and the potential limiting steps are shown to be \({}^{*}+{{{{{\rm{C}}}}}}{{{{{{\rm{O}}}}}}}_{2}\to {}^{*}{{{{{\rm{C}}}}}}{{{{{\rm{O}}}}}}{{{{{{\rm{O}}}}}}}^{-}\) for CuN 4 C 4 , \({}^{*}{{{{{\rm{CO}}}}}}\to {}^{*}{{{{{\rm{CHO}}}}}}\) for CuN 3 C 3 and CuN 2 C 2 (Supplementary Fig. 47 ). The magnitudes of the corresponding theoretical limiting free-energy differences ( ΔG L ) are summarised in Supplementary Fig. 47 . While the three distinctly coordinated catalysts exhibit a flipped volcano relationship for CO and formate activities, the predicted HER and CH 4 /CH 3 OH activities are simultaneously enhanced by lowering the local symmetry via introducing N vacancy. In comparison to the highly symmetrical CuN 4 C 4 , it leads to a much lower ΔG L (0.23 eV) for the formate pathway than the CO (0.68 eV), CH 4 /CH 3 OH (0.78 eV) and HER (1.01 eV) pathways in the local symmetry-broken CuN 3 C 3 . But, this tendency is reversed by more N vacancies in CuN 2 C 2 which exhibits a preference to the HER pathway. The high selectivity for CO 2 conversion to formate in CuN 3 C 3 can be also appreciated from the large difference between the ΔG L for CO 2 reduction and HER. The probability for C 2 products generation was also considered by examining the first C–C coupling of two *CO species that is crucial for the formation of C 2 products (Supplementary Fig. 47 ). This step is found to have a large ΔG L (1.79 eV on CuN 4 C 4 and 1.67 eV on CuN 3 C 3 ), indicating a formidable C–C coupling of *CO species for the generation of C 2 products. Thus, the HCOOH production is thermodynamically preferred than the generation of other C 1 and C 2 products and H 2 on the CuN 3 C 3 structure at zero electrode potential. Because the electric field can interact with intermediates with a substantial dipole moment and/or polarizability [49] , [50] , [51] , we further examined the effects of interfacial electric field and pH on the adsorbate bindings on different CuN x C y structures (Supplementary Table 7 ). A significant response of the adsorbate bonding strength to the electric field effects is revealed in Fig. 4a and Supplementary Fig. 48 . Then, an applied potential of −0.80 V vs. RHE and pH = 7.3 is considered and it leads to a remarkable decrease of the free energy for the adsorbates (Fig. 4b–e , Supplementary Figs. 49 and 50 ), which indicates more stabilised intermediates and decreased endothermicity for the reaction steps. On the CuN 3 C 3 structure, the potential limiting steps for formate and CO productions are shifted to \({}^{*}{{{{{\rm{OC}}}}}}{{{{{\rm{O}}}}}}^{-} \to {}^{*}{{{{{\rm{OCHO}}}}}}\) and CO desorption, respectively (Fig. 4b ), and it produces a considerably lower limiting free-energy difference ( ΔG L ) of −0.03 eV for the formate pathway (Fig. 4e ), which is in contrast to the comparable ΔG L between the HER (0.51 eV), CO (0.63 eV) and CH 4 /CH 3 OH (0.51 eV) pathways, indicating a strong preference to the formate production. By contrast, a much higher ΔG L of 0.62 eV is shown for the formate pathway on the CuN 4 C 4 structure. This prediction agrees well with the impressively higher FE for CO 2 RR-to-formate on PSB-CuN 3 catalyst than on PS-CuN 4 catalyst over similar potential range (see Fig. 3 ). CuN 2 C 2 exhibits an extremely strong preference to the HER pathway with a ΔG L of −0.68 eV. Similar potential dependence is obtained at an applied potential of −0.40 V vs. RHE (Supplementary Table 7 ). All in all, the adsorbate energies corrected for the electric field and pH effects strongly support the highest activity and selectivity toward formate in the local symmetry-broken CuN 3 C 3 moiety. Fig. 4: First-principles calculations and operando XAFS characterisation on PSB-CuN 3 catalysing CO 2 RR. a Electric field effects on the adsorbate bindings on the CuN 3 C 3 structure. b – d Gibbs free-energy diagrams for CO 2 electroreduction to CO, HCOOH, H 2 , CH 4 and CH 3 OH on CuN 3 C 3 structure. The highlights indicate the potential limiting steps. e Magnitudes of the theoretical limiting free-energy differences ( ΔG L ) for CO, HCOOH, H 2 and CH 4 /CH 3 OH productions. f Differential charge density and projected density of states for the Cu centre and the bound O atom in the adsorbed *OCHO intermediates supported on CuN 3 C 3 structure. White, grey, blue, red and cyan balls represent H, C, N, O and Cu atoms, respectively. The black dashed line represents the Femi energy level. g Adsorption free energies of ΔG *OCO − , ΔG *COO − , ΔG *OCHO , ΔG *COOH and ΔG *H vs. the descriptor φ . h Thermodynamic relations (volcano) lines for the H 2 , CO and HCOOH productions as a function of the descriptor φ . i Fourier-transformed magnitudes of operando Cu K -edge EXAFS spectra for PSB-CuN 3 recorded at various applied potentials vs. RHE in 0.5 M KHCO 3 aqueous solution. a.u., arbitrary units. Full size image To understand why the modified electronic structure in PSB-CuN 3 catalyst is in favour of CO 2 reduction toward formate, the projected density of states for the adsorbed intermediates of *COO − and *OCO − were obtained. Supplementary Fig. 51 shows the overlap degree between Cu- d and O- p orbitals is generally larger than that between Cu- d and C- p orbitals on each CuN x C y structure, thus indicating a stronger binding of *OCO − than *COO − . For *OCO − , the overlap degree between Cu- d and O- p orbitals in CuN 3 C 3 and CuN 2 C 2 is obviously increased as compared to CuN 4 C 4 . However, the binding of the intermediates in CuN 2 C 2 is so strong that the potential limiting step shifts to the formate desorption. It suggests that the local symmetry-broken CuN 3 C 3 can produce a suitable overlap degree between the Cu- d and O- p orbitals, which can result in a neither strong nor weak binding of the intermediates. Thus, those results unveil that the highest activity and selectivity toward formate in the local symmetry-broken CuN 3 C 3 moiety is strongly correlated with its unusual coordination environment, in good agreement with the experimentally detected excellent activity of the PSB-CuN 3 catalyst in electrochemical CO 2 reduction (Fig. 3 ). The intrinsic coordination characteristics of the active CuN x centres that dominate the adsorbate binding strength and activity are explored. Breaking of the local D 4 h symmetry to create planar-like CuN 3 and CuN 2 moieties with lower local C 2 v symmetry leads to charge redistribution (Fig. 4f ) and increased attractive interactions for the intermediates (Fig. 4b–e ). The charge redistribution is first manifested as an obvious upshift of the d -band centre of Cu atom in energy relative to the Fermi level from CuN 4 to CuN 3 moiety, but this tendency is reversed by a dramatic downshift of the d -band centre in CuN 2 moiety (Supplementary Fig. 52a ). This anomaly leads to the widely used d -band centre model cannot correlate with the increased adsorbate binding strength and activity (Supplementary Fig. 52b, c ), which stems from the enhanced dsp orbitals hybridisation near the Fermi level in local symmetry-broken CuN x moieties (Supplementary Fig. 53 ) as also indicated by experimental XANES results. By contrast, the total electron transfer from Cu and the work function appear to be dominated by the coordination number of nearest-neighbour N atoms (denoted as n N , Supplementary Fig. 54a–c ), which matches well with the valence state change obtained by XANES. In addition, approximate linear relationships are observed when n N is plotted against adsorption energies and limiting free-energy differences for different intermediates (Supplementary Fig. 54d, e ), which suggests that n N can be a significant factor of the descriptor [52] . Besides, it is noted that angular distortion has been widely used to describe the stereochemical activity of ns [2] electron pairs in metal halide perovskites ABX 3 [53] . It suggests that the angle distortion between neighbouring Cu–N bonds in the present work can further modify the charge redistribution and binding affinity, and we add it as an additional factor to modify the descriptor as follows: 
    φ=n_N×(1-1/n_a∑_{i=1}^n_a|90-α_i/90|)
 (1) where n N is the number of nearest-neighbour N atoms, α i is the N–Cu–N bond angle between neighbouring Cu–N bonds and n a is the number of the N–Cu–N bond angles. As shown in Fig. 4g , Supplementary Fig. 55 and Supplementary Table 8 , excellent linearity is obtained between φ and the adsorption energies for *COO − , *OCO − , *COOH, *OCHO and *H. It means that a decrease in φ corresponds to an enhancement in binding strength, which particularly causes a tighter binding of *COO − , *OCO − , *COOH, *OCHO and *H. This can be attributed to the adoption of a peculiar slant adsorption way (instead of the conventional top-site way, see Fig. 4f ) of *OCHO intermediate on the CuN x centres with the successive introduction of N vacancy. It leads to an unusual coupling between the in-plane and out-of-plane 3 d , 4 s and 4 p orbitals of the Cu centre and the 2 s and 2 p orbitals of the bonded O atom of intermediates (Fig. 4f , Supplementary Figs. 56 – 58 ). It suggests that the orbital coupling degree and binding affinity between the Cu centre and the intermediates is directly correlated with the local geometric symmetry breaking of the surrounding N atoms (Supplementary Note 3 ). Figure 4h shows the theoretical limiting free-energy differences versus the descriptor φ . While a good linearity with different slopes is shown for H 2 production, a flipped volcano relationship is revealed for CO, formate and CH 4 /CH 3 OH productions, with the CuN 3 moiety lying at bottom of the volcano. The relative order of activity and selectivity from the theoretical prediction reproduces well the experiment data (Fig. 3 ), thus validating our descriptor φ . Hence, the local coordination symmetry breaking, which is quantified as a combination of nearest-neighbour coordination number and bond angle distortion, can serve as a universal descriptor to evaluate the activity of graphene-based single Cu catalysts towards CO 2 RR. The dynamic processes for CO 2 adsorption and activation towards highly selective production of formate on PSB-CuN 3 were further investigated by experimental Cu K -edge XAFS spectroscopy under operando conditions (Fig. 4i , Supplementary Figs. 59 – 66 , Supplementary Table 1 ). The XANES spectra display that the Cu K -edge of pristine PSB-CuN 3 initially shifts to higher energy and the intensity of the shoulder peak D also increases when immersing in CO 2 -saturated 0.5 M KHCO 3 solution under open-circuit potential (OCP) bias (Supplementary Fig. 59a ). This indicates an increased oxidation state for the Cu sites, which is caused by the charge transferred from low-valent Cu 1+ to CO 2 molecule to form CO 2 δ + species. This assumption is consistent with a slight contraction of the first major peak from 1.60 Å to 1.58 Å as well as an elongation of the second satellite peak from 2.20 Å to 2.26 Å in EXAFS-FT under OCP bias (Fig. 4i ). It reflects an additional contribution from the Cu–O bond of the dynamically adsorbed CO 2 molecular. During CO 2 reduction at −0.5 V and −0.8 V vs. RHE, the Cu K -edge XANES shows a shift back to lower energy without obvious profile change, which indicates the adoption of a low oxidation state for the Cu sites during the catalytic stage, corroborating the high activation ability of CuN 3 C 3 centres for CO 2 reduction. Meanwhile, the first two peaks in EXAFS-FT, which now consists of the Cu–N bonds and the Cu–O/C bonds from the reaction intermediates (e.g., *OCO − , *OCHO), demonstrates a continuous shift to shorter length and an increase in intensity (Fig. 4i ), corresponding to a contraction of Cu–N/O/C bonds with decreased bond disorder. When the applied potential returns to OCP, both XANES and EXAFS-FT reverse to the initial OCP state. Further quantitative EXAFS curve-fitting analysis reveals a decrease in Cu-N/O/C interatomic distances as well as an increase in coordination numbers during the operating process (Supplementary Fig. 63 and Supplementary Table 1 ). Similar evolution behaviours for the electronic and atomic structures of the metal centres under the catalytic conditions have also been observed in single-Ni-atom catalyst for CO 2 reduction to CO [54] . Here, the above phenomena consolidate a tighter binding of the reaction intermediates (e.g., *OCO − , *OCHO) under the catalytic conditions, which is suggested to be responsible for the high catalytic activity and selectivity of the PSB-CuN 3 . At the same time, attenuated total reflectance surface-enhanced infra-red absorption spectroscopy (ATR-SEIRAS) was used to probe the reaction intermediates on PSB-CuN 3 (Supplementary Fig. 67 ). When the applied potential is more negative than −0.8 V vs. RHE, the obvious peak at ~1620 cm –1 exhibits a pronounced rise and red shift, which can be ascribed to the asymmetrical O–C–O stretching band of dissolved formate. Additionally, two broad bands appeared between 1450 and 1350 cm –1 , and they can be assigned to the symmetrical O–C–O stretching mode of bridge-bonded formate and the C–OH vibration of desorbed formate molecules, respectively [55] . No signal of *COO − /*COOH was detected. These findings evidence the preferred formation of *OCO − /*OCHO intermediates bonded to the PSB-CuN 3 catalyst via O. The impact on the catalytic and structural stability from N coordination number variation is investigated (See detailed discussion in Supplementary Note 4 ). While PSB-CuN 3 shows better electrocatalytic stability than PS-CuN 4 in both H-cell and flow cell under the same applied potential, the detailed operando and postmortem XAFS with AC-HAADF-STEM characterisations revealed a structural reconstruction occurs on both PSB-CuN 3 and PS-CuN 4 during CO 2 reduction. Compared with PS-CuN 4 with high valence Cu 2+ , the structure change of low-valent Cu 1+ PSB-CuN 3 is slight. And, the structural evolution process of PSB-CuN 3 is reversible and no atoms aggregation can be observed after CO 2 electrocatalysis. On contrary, the dramatic structural reconstruction of PS-CuN 4 leads to an irreversible aggregation of fractional Cu atoms. Therefore, the electrochemical stability of PSB-CuN 3 is better than that of PS-CuN 4 , consistent with previous works that the low-valent Ni 1+ single-atom catalysts showed no reconstruction into nanoparticles for CO 2 RR to CO [54] , but the high-valent Cu 2+ single-atom catalysts reconstructed to nanoparticles in the electrochemical reduction of nitrate to ammonia [56] and electrocatalytic oxygen reduction [57] . In summary, the local planar-symmetry-broken PSB-CuN 3 is successfully prepared by a simple and facile method, and further used as the electrocatalysts for CO 2 RR. Significantly, the as-prepared PSB-CuN 3 catalyst exhibits extremely high electrocatalytic activity and catalytic stability in both H-cell and flow cell systems, superior to the highly symmetrical PS-CuN 4 and comparable to recently best-reported CO2RR-to-HCOO − catalysts. By combining ex-situ/operando EXAFS, XANES and ATR-SEIRAS analyses with theoretical calculations, we unambiguously unveiled that the high catalytic performance for formate production originates from the intrinsic local symmetry breaking from the planar-like D 4 h to C 2 v configuration in PSB-CuN 3 , such that an unconventional dsp hybridisation is emerged. With this anomaly, the catalytic activities are unconformable to the widely used d -band centre theory, whereas the local environment of the metal centre including coordination number and geometric distortion is identified as a newly universal descriptor to the intermediate adsorption and thus catalytic activities for H 2 /CO/HCOOH/CH 4 /CH 3 OH productions in graphene-based SACs. Our study provides a universal and efficient guideline for the rational design and accurate modulation of the active centre’s local symmetry in nonprecious metal SACs for diverse CO 2 RR applications at the atomic scale. Chemicals CuCl 2 ·6H 2 O (99.99% AR grade) was bought from Alfa Aesar. Nafion solution (5 wt%), natural graphite flakes (100 mesh), ammonia solution (~30%) and KHCO 3 (99.95%) were obtained from Sigma Aldrich. All chemicals were used directly without further purification. The ultrapure water (18 MΩ) used in the experiments was supplied by a Millipore System (Millipore Q). Synthesis of PSB-CuN 3 and PS-CuN 4 Graphene oxide (GO) was first synthesised by a modified Hummers’ method [58] . Then, NH 4 OH solution (0.5 mL) was added dropwise to a GO aqueous suspension (5 mL, 2 mg mL −1 ) and stirred for 20 min. The mixed suspension was transferred to a Teflon vessel at 70 °C for 5 h under airtight conditions. After cooling and six times washing using water, the purified AGNs were obtained. Subsequently, 80 μL CuCl 2 ·6H 2 O (3 mg mL −1 ) was added to the well-dispersed AGNs solution under stirring for 1 h. The purified samples were subsequently transferred into a freeze-drying vessel, which had been set at the temperature of −53 °C and vacuum pressure of −30 Pa. After being freeze-dried, the Cu 2+ -containing AGNs, together with small amounts (≈1 wt%) of thermally reduced (300 °C for 1 h in Ar) graphene as catalysts, were sealed in an Ar gas-protected glass vial and then undergo a microwave process (microwave digestion workstation XH-800C) under 1000 W for 5 s [59] . PSB-CuN 3 was collected after a cooling period for 20 min. For comparison, PB-CuN 4 was synthesised by the pyrolysis of Cu 2+ -containing AGNs in an Ar/NH 3 mixed atmosphere according to the reported method [17] . Physical characterisations XRD patterns were collected by using a Bruker D8 Advance X-ray powder diffractometer with a Cu K α irradiation source (λ = 1.5406 Å), and a self-calibration process was performed with a SiO 2 internal standard sample prior to target measurement. The sizes and morphologies of the samples were first recorded using a Hitachi H-800 transmission electron microscope. Then, the high-resolution STEM and elemental mappings were carried out on a JEOL JEM-2100F with an electron acceleration energy of 200 kV. A JEM-ARM200F transmission electron microscope operated at 200 keV, equipped with a probe spherical aberration corrector, was used to obtain HAADF-STEM images of the samples. All TEM/STEM samples were prepared by depositing a tiny amount of the samples onto a molybdenum (Mo) grid. Quantitative analysis of metal loading was carried out using inductively coupled plasma atomic emission spectroscopy (TJA RADIAL IRIS 1000 ICP-AES). XPS spectra were performed by a Thermo Scientific K-Alpha spectrometer using a monochromatic Al K α radiation, where the analysis chamber was 1.5 × 10 −9 mbar and the X-ray spot was ~500 μm. The C 1 s peak for adventitious hydrocarbons at 284.8 eV was used for binding energy calibration. Raman measurements were conducted on a Renishaw Microscope System RM2000 with a Renishaw spectrometer of 532 nm. The N 2 adsorption/desorption curve was performed at 77 K using a Quadrasorb SI (Quantachrome, USA) surface area analyser. Electrochemical measurements The electrochemical measurements were performed on a CHI 760e electrochemical workstation in a three-electrode configuration cell using an as-prepared electrode as the working electrode, platinum wire as the counter electrode and Ag/AgCl (saturated KCl) as the reference electrode in 0.5 M KHCO 3 aqueous electrolyte. Nafion117 membrane was inserted between the cathodic chamber and anodic chamber of H-type cell. The catalyst inks were prepared by a mixture of catalyst (5 mg), water (240 μL), isopropanol (750 μL) and 5% Nafion solution (10 μL), followed by ultrasonication for 4 h. An aliquot of 0.1 mL of the catalyst ink was deposited onto carbon paper (HCP120, Shanghai Hesen Electric Co., Ltd) and allowed to dry in air, giving a catalyst loading of 0.5 mg cm −2 . Before the measurement, the 0.5 M KHCO 3 aqueous solution (pH = 7.3) was purged by bubbling Ar for 30 min and then switched to CO 2 until saturation. The LSV curves were conducted at a scan rate of 10 mV/s with continuous bubbling CO 2 . For comparison, cyclic voltammetry curves tested in an Ar (99.99%)-saturated electrolyte were also obtained. All potentials were converted to the RHE scale according to the standard Nernst equation ( \({{{{{{\rm{E}}}}}}}_{{{{{{\rm{RHE}}}}}}}={{{{{{\rm{E}}}}}}}_{{{{{{\rm{Ag}}}}}}/{{{{{\rm{AgCl}}}}}}}+0.0591\times {{{{{\rm{pH}}}}}}+0.197{{{{{\rm{V}}}}}}\) ). All current densities were normalised to the geometrical area of electrode (1 × 1 cm 2 ). The gas products of CO 2 RR were checked by online gas chromatography (GC, Supplementary Fig. 33 ). The 1 H NMR spectroscopy was used to analyse and quantify the products in the liquid phase (Supplementary Fig. 34 ). Samples were prepared by mixing DMSO and electrolyte aliquots. All the potentials were reported vs. RHE and manually corrected by 100% iR compensation, which was obtained through electrochemical impedance spectroscopy (Supplementary Fig. 30 and Supplementary Table 9 ). EIS measurements were conducted at 25 °C using an H-type cell (consisting of two independent anode and cathode chambers separated by a nafion membrane) and a CHI 760e electrochemical workstation. Platinum wire served as the counter electrode, while Ag/AgCl (saturated with KCl) was employed as the reference electrode. The EIS measurement was carried out under open-circuit voltage, and the frequency setting range was from low frequency 1 Hz to high frequency 100,000 Hz. The amplitude was set as 0.005 V. For the flow cell study, catalyst inks were air-brushed onto a gas diffusion layer (GDL) as the cathode electrode with a mass loading of ~0.6 mg cm −2 . IrO 2 was used as the counter electrode. The IrO 2 catalyst ink was prepared by a mixture of commercial IrO 2 powder (5 mg), water (240 μL), isopropanol (750 μL) and 5% Nafion solution (10 μL), followed by ultrasonication for 4 h. Then, IrO 2 catalyst (0.7 mg/cm 2 ) was loaded onto the GDL as anode. Electrolyte was pumped by a syringe pump (PHD 2000, Harvard Apparatus) over the cathode GDL at a constant flow rate of 10 standard cubic centimetres per minute (sccm). High-purity CO 2 gas flowed at a rate of 30 sccm behind the cathode GDL controlled by a mass flow controller (CS200, Beijing Sevenstar flow). Polarisation curves of all studied electrodes are performed at a sweeping potential between 0 and −1.2 V vs. RHE (all potentials reported here were based on RHE) with a scan rate of 10 mV s −1 . Gas product analysis Gas products from the cathodic compartment during the electrochemical reactions were analysed using a GC-2014 (Shimadzu) equipped with a BID detector and ShinCarbon ST100/120 packed column. High-purity helium (99.9999%) was used as the carrier gas. The FEs of the gas products were calculated by using the concentrations (ppm) detected by the GC as follows (CO products are selected as an example): 
    FE_CO(%)=Q_CO/Q_total× 100%=(ν/60s/min) ×(y/22400cm^3/mol)× N× F× 100%/j
 (2) where ν is gas flow rate measured by a flowmeter at the exit of the cell at room temperature, y is the measured volume concentration of product, N is the number of electrons required to form a molecule of gas product, F and j are the Faraday constant (96,500 C mol −1 ) and the recorded current, respectively. Liquid product analysis Liquid products were analysed by using a 400 MHz NMR spectrometer (Bruker), with DMSO as internal standards. The calibration curve was made by measuring standard solutions of formate. The FEs of liquid products were calculated as follows: 
    FE_HCOO^-(%)=Q_HCOO^-/Q_total× 100%=n_HCOO^-× N× F× 100%/j× t
 (3) where n HCOO− is the measured amount of formate in the cathodic compartment and t is the reaction time. The HCOO − partial current density at different potentials was calculated by multiplying the overall geometric current density and its corresponding FE. Turnover Frequency (TOF, h −1 ) for the CO 2 electroredution to formate was evaluated based on the 2-electron pathway: 
    TOF=I_product/NF/m_cat× w/M_metal× 3600
 (4) where I product is the partial current for formate, N is the number of electrons transferred for product formation, F is the Faraday constant (96,500 C mol −1 ), m cat is the catalyst mass in the electrode, w is the metal loading in the catalyst and M metal is the atomic mass of Cu (63.5 g mol −1 ). Soft XAS measurements Soft C, N K -edge and Cu L 3,2 -edge X-ray absorption spectra were measured at BL12B station of Hefei National Synchrotron Radiation Laboratory in the total electron yield mode by collecting the sample drain current under a vacuum better than 10 −7 Pa. Ex-situ and operando XAFS measurements Hard X-ray absorption spectra at Cu K -edge were acquired under ambient conditions in fluorescence mode using Si(111) double-crystal monochromators at 1W1B and 4B9A beamlines of Beijing Synchrotron Radiation Facility (BSRF, operated at 2.5 GeV with a maximum current of 250 mA). The incident and fluorescence X-ray intensities were monitored by using standard N 2 -filled ion chambers and air-filled Lytle-type detector, respectively. A home-made cell collected to a computer-controlled electrochemical analyser was used for the operando XAFS experiments, which were operated under identical conditions as the electrochemical measurements. A catalyst-modified carbon paper was used as working electrode, Pt wire as counter electrode and Ag/AgCl (KCl-saturated) electrode as the reference electrode. CO 2 -saturated 0.5 M aqueous KHCO 3 was used as electrolytes. Operando XAFS spectra were recorded at different potentials to monitor the structural evolutions of the catalysts. XAFS data analysis The XAFS raw data were background-subtracted, normalised and Fourier-transformed by the standard procedures with the ATHENA programme [44] , [60] , and least-squares curve-fitting analysis of the EXAFS χ (k) data was carried out using the ARTEMIS programme based on the standard EXAFS equation. All fits were performed in the R space with k -weight of 2. The best-fit results are shown in Supplementary Figs. 13 – 17 with the fitting parameter values listed in Supplementary Table 1 . The Cu K - and L -edge theoretical XANES calculations were carried out with the FDMNES code in the framework of real-space full multiple-scattering (FMS) scheme using Muffin-tin approximation for the potential [43] , [61] , [62] . The energy-dependent exchange-correlation potential was calculated in the real Hedin–Lundqvist scheme, and then the spectra was convoluted using a Lorentzian function with an energy-dependent width to account for the broadening due both to the core–hole width and to the final state width. The CuN x C y moieties were built based on the graphene-enclosed MN 4 C 4 structural motif (Supplementary Fig. 21 ), which can be regarded as a single Cu atom occupying the divacancy in the graphene lattice with coordination to four pyridinic Ns included in six-member rings. Satisfactory convergence for the cluster sizes had been achieved. Operando ATR-SEIRAS Operando ATR-SEIRAS was performed on a Nicolet iS20 spectrometer equipped with a VeeMax III (PIKE technologies) accessory and an HgCdTe (MCT) detector cooled with liquid nitrogen. The electrochemical test was conducted in a custom-made three-electrode electrochemical single cell. A Pt wire and a saturated Ag/AgCl were used as the counter and reference electrodes, respectively. A fixed-angel Si prism (60°) coated with Au thin layer was used to load catalysts and serve as the working electrode. The operando ATR-SEIRAS spectra were recorded by varying the potential in CO 2 -saturated 0.50 M KHCO 3 . The spectrum recorded at the initial potential of 0 V was used for the background subtraction. Computational method and models The first-principles calculations including structural and electronic performances were carried out in the framework of density functional theory (DFT) as implemented in the Cambridge Sequential Total Energy Package (CASTEP) [63] . The exchange-correlation functional under the generalised gradient approximation (GGA) with norm-conserving pseudopotentials and Perdew–Burke–Ernzerhof functional was adopted to describe the electron-electron interaction [64] . The spin polarisation was considered [52] . The DFT-D2 method of Grimme for the Van der Waals correction was used [65] . An energy cutoff of 750 eV and a k -point sampling set of 5 × 5 × 1 were tested to be converged. A force tolerance of 0.01 eV Å −1 , energy tolerance of 5.0 × 10 −7 eV per atom and maximum displacement of 5.0 × 10 −4 Å were adopted. The surfaces of the structures were built with a vacuum space of 20 Å along the z-direction, which is enough to avoid interaction between the two neighbouring images. The effect of water was considered by using the implicit solvent model with the dielectric constant of 78.54 for water molecule. The structure models were built with a vacuum space of 20 Å along the z-direction, which is enough to avoid interaction between the two neighbouring images. Then the intermediates for CO, HCOOH, H 2 , CH 4 , CH 3 OH and C 2 products were adsorbed on the active centres. All the atoms were relaxed to release the internal stress of systems. In addition, an electric field was applied to consider its effect on the binding geometry and energy of the adsorbates. The formation energy of the active centres was estimated by: 
    ΔE_f=E_sys-n_C*μ_C-n_N*μ_N-n_H*μ_H-μ_Cu
 (5) where E sys was the total energy of each system; n C ,n N and n H denoted the amounts of C, N and H atoms in each system; μ C , μ N and μ H were the chemical potentials of C, N and H atoms, denoting the energy of per C, N and H atom in graphite, N 2 gas and H 2 gas. The adsorption energy Δ E ads of each intermediate on the surface of substrates was defined as: 
    ΔE_ads=E_inter^*-(E_^*+E_inter)
 (6) where the subscripts inter* and * denoted the adsorption of intermediate on substrates and the bare substrates, E inter denoted the energy of intermediate. The Gibbs free energy (Δ G ) of each chemical reaction without external electric field (i.e., E = 0) was calculated by: 
    ΔG_ads^E=0=ΔE_ads^E=0+ΔZPE-TΔ S
 (7) where Δ E ads , Δ ZPE , T and Δ S denoted the calculated total energy, zero point energy, temperature and entropy, respectively. Then, the energy was corrected for the RHE scale and electric field by [49] , [50] : 
    ΔG_ads=ΔG_ads^E=0+μ E-αE^2/2-neU_RHE
 (8) where E was the external electric field, ne was the amount of proton–electron pairs transferred in each chemical reaction, U RHE was the applied potential vs. RHE. The values of μ and α were acquired from the second-order polynomial fitting for the energy of each adsorbate across the range of electric fields (see Supplementary Fig. 48 ). The external electric field was pH-dependent on an RHE scale and estimated by: 
    E=C_H(.U_RHE-κ_BT  ln(10)×pH-U_PZC/ϵϵ_0
 (9) where C H = 20 μF cm −2 refers to Helmholtz capacitance for archetypical carbon material [66] , ϵ 0 refers to vacuum permittivity (8.85 ×10 −12 F m −1 ), ϵ = 2 refers to dielectric constant of water near a surface (unitless), k B is the Boltzmann constant, T = 300 K and pH = 7.3 is kept consistent with experimental conditions, U PZC = 0.22 V refers to the potential at the point of zero charge (PZC) vs. SHE, which was measured by differential capacitance curves using impedance methods [67] . Five electrochemical reaction pathways were considered [47] , [48] , [68] : (I) For formate production, 
    ^*+CO_2+e^-→^*O^-OC
 (10) 
    ^*OCO^-+H^+→^*OCHO
 (11) 
    ^*OCHO+(H^++e^-)→^*HCOOH
 (12) 
    ^*HCOOH→^* +HCOOH
 (13) (II) For formate production, 
    ^*+(H^++e^-)→^*H
 (14) 
    ^*H+CO_2→^*OCHO
 (15) 
    ^*OCHO+(H^++e^-)→^*HCOOH
 (16) 
    ^*HCOOH→^* +HCOOH
 (17) (III) For CO production, 
    ^*+CO_2+e^-→^*O^-CO
 (18) 
    ^*O^-CO+H^+→^*COOH
 (19) 
    ^*COOH+(H^++e^-)→^*CO+H_2O
 (20) 
    ^*CO→^* +CO
 (21) (IV) For CO production, 
    ^*+(H^++e^-)→^*H
 (22) 
    ^*H+CO_2→^*COOH
 (23) 
    ^*COOH+(H^++e^-)→^*CO+H_2O
 (24) 
    ^*CO→^* +CO
 (25) (V) For hydrogen evolution reaction, 
    ^*+(H^++e^-)→^*H
 (26) 
    ^*+(H^++e^-)→^*H
 (27) The electrochemical reaction steps for CH 4 , CH 3 OH and C 2 productions were referred to in the published works [48] , [60] .